Nanoscale determination of the mass enhancement factor in the lightly doped bulk insulator lead selenide Bismuth chalcogenides and lead telluride/selenide alloys exhibit exceptional thermoelectric properties that could be harnessed for power generation and device applications. Since phonons play a significant role in achieving these desired properties, quantifying the interaction between phonons and electrons, which is encoded in the Eliashberg function of a material, is of immense importance. However, its precise extraction has in part been limited due to the lack of local experimental probes. Here we construct a method to directly extract the Eliashberg function using Landau level spectroscopy, and demonstrate its applicability to lightly doped thermoelectric bulk insulator PbSe. In addition to its high energy resolution only limited by thermal broadening, this novel experimental method could be used to detect variations in mass enhancement factor at the nanoscale level. This opens up a new pathway for investigating the local effects of doping and strain on the mass enhancement factor. The effects of interactions between electrons and phonons can be ubiquitously observed in systems ranging from simple metals [1] , to more exotic materials such as graphene [2] , [3] , high-temperature superconductors [4] , [5] , [6] , [7] , [8] , [9] and topological insulators [10] , [11] , [12] , [13] , [14] , [15] , [16] . In general, electron–phonon interactions give rise to quasiparticles of decreased mobility and increased effective mass. This process is theoretically captured by the Eliashberg function α 2 F( ω ; k , E ) (ref. 17 ), which encodes the scattering of quasiparticles by coupling to a bosonic mode of frequency ω . The Eliashberg function is related to the complex self-energy of the system (Σ( k , E )) (ref. 17 ), an experimentally accessible quantity that contains both the quasiparticle energy shift due to interactions (Σ′( k , E )=Re{Σ( k , E )}) and its lifetime (Σ″( k , E )=Im{Σ( k , E )}). Σ′( k , E ) and Σ″( k , E ) are related to one another by Kramers–Kronig relations, so knowing only one of them should, in principle, be sufficient to determine the total self-energy Σ( k , E ), and thus the Eliashberg function itself [18] . Since many fundamental properties, such as the electron mass enhancement factor ( λ ), can be calculated from the Eliashberg function, its precise experimental determination is of immense importance. In topological materials, there are clear instances where electron–phonon coupling (EPC) has measurable physical effects [10] , [19] . Although relatively well described within the framework of non-interacting Dirac theory, surface state Dirac fermions in topological materials are experimentally found to interact with lattice excitations [10] , [11] , [12] , [13] , [14] , [15] , [16] , leading to the renormalization of the underlying surface state band structure. The role and magnitude of this interaction are still under debate, as vastly different results have been obtained not only across different techniques, but also using the same experimental probe on nominally identical compounds [13] , [14] . For example, the measured λ in a typical three-dimensional topological insulator Bi 2 Se 3 is found to range from as low as λ ~0.17 (ref. 13 ) (measured at 20 K) to λ ~3 (ref. 14 ) (measured at 7 K) in recent laser-based angle-resolved photoemission spectroscopy (ARPES) studies reported by two different groups. Careful analysis by Howard and El-Batanouny showed that different acquisition temperatures (7 K vs 20 K) would account for some of the discrepancy, but only less than a factor of 2 between the two studies [20] . Possible reasons for this discrepancy may be the resolution of the technique or the inability to detect the 3-meV phonon peak in ref. 13 , which was reported by Kondo et al . [14] Another contributing factor might lie in the intrinsic structural inhomogeneity (local chemical potential variation, step-edges, defects, strain/stress, and so on) present on the surface of these materials, either as an inevitable consequence of the cleavage process or the varying sample quality. Thus, developing a high-resolution technique for local determination of EPC on nanometre length scales with simultaneous imaging of the surface and the local density of states would be of tremendous importance not only for obtaining λ with a measure of reliability, but also for a deeper understanding of the factors affecting EPC, and ultimately for measuring the Eliashberg function for interacting systems such as superconductors or charge density wave materials where the EPC plays an important role in determining their ground state. To illustrate subtle self-energy effects present due to the interaction of phonons and electrons, let us use a single electronic band crossing the Fermi level as an example ( Fig. 1 ). In the absence of EPC, this band is expected to smoothly cross the Fermi level. However, when EPC is turned on, an antisymmetric kink develops in the dispersion near the Fermi level. To reliably extract this band renormalization, high-resolution experimental determination of the electronic band structure is crucial. Scanning tunnelling microscopy (STM) has been successfully applied to nanoscale band structure mapping using either the method of quasiparticle interference (QPI) [21] , [22] or Landau level (LL) spectroscopy [23] , [24] , [25] . In relatively simple systems such as Ag(111), QPI imaging has proven effective for the detection of small kinks in the electronic dispersion, which allowed the approximation of the electron mass enhancement λ (ref. 26 ). Applying the same technique to Fe-based high-temperature superconductors has revealed the momentum–space anisotropy in self-energy likely originating from antiferromagnetic spin fluctuations [9] . Therefore, this method could naturally be extended to other materials. However, it cannot be used in many three-dimensional topological materials as the fundamental nature of the topological surface states prohibits quasiparticle backscattering [27] and therefore prevents the observation of QPI in the desired energy range [28] , [29] . Furthermore, the extracted band structure from QPI measurements is often noisier [25] , requires longer time acquisition and provides lower energy resolution compared with the band mapping using LL spectroscopy. 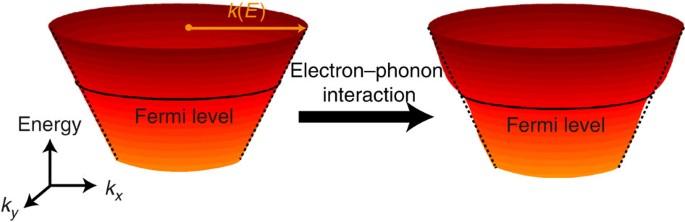Figure 1: Schematic of the EPC effect on band structure of topological materials. In the absence of EPC (left), the Dirac SS band smoothly crosses the Fermi level. However, when EPC is turned on (right), electronic density of states gets renormalized, resulting in a ‘kink’ in the SS dispersion near the Fermi level. Figure 1: Schematic of the EPC effect on band structure of topological materials. In the absence of EPC (left), the Dirac SS band smoothly crosses the Fermi level. However, when EPC is turned on (right), electronic density of states gets renormalized, resulting in a ‘kink’ in the SS dispersion near the Fermi level. Full size image In the following, we will describe the first utilization of LL band mapping to extract the self-energy, the Eliashberg function and λ in a trivial bulk insulator Pb 1- x Sn x Se with x ~0.09. Surface characterization Single crystals of Pb 1− x Sn x Se are prepared using the self-selecting vapour growth method, cleaved at ~77 K in ultra-high-vacuum, and immediately inserted into the STM where they are held at 4 K during data acquisition. Although the process of cleaving can result in multiple surface step-edges and even distinct cleavage planes, we are able to find microscopically large, atomically flat regions characterized to be the (001) surface based on the square atomic lattice observed in STM topographs ( Fig. 2a ). The average conductance d I/ d V spectrum, which is directly proportional to the local density of states, exhibits a clear gap of ~50 meV ( Fig. 2b ), confirming that this composition would be a band insulator without the intrinsic doping due to defects that moves the Fermi energy into the conduction band. Although Pb 1- x Sn x Se is non-topological at the alloying composition studied, it hosts distinct trivial surface states that can be observed and studied using STM [30] . We note here that the gap measured by us sets a lower limit for the band gap; the actual value may be larger but masked due to the surface state. We proceed to describe the utilization of LL spectroscopy to map an electronic band crossing the Fermi level for the purposes of quantifying many-body interactions. 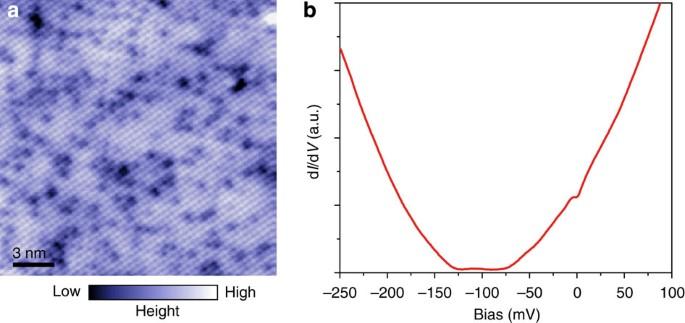Figure 2: Typical STM topograph and dI/dVspectrum. (a) Typical STM topograph of the (001) surface showing a clear square lattice. (b) Average dI/dVspectrum obtained over the region of the sample ina, showing an integrated density of states gap of ~50 meV that sets a minimum value for the band gap at this composition. Setup conditions in: (a)Iset=10 pA,Vset=−100 mV; (b)Iset=100 pA,Vset=−100 mV. Figure 2: Typical STM topograph and d I/ d V spectrum. ( a ) Typical STM topograph of the (001) surface showing a clear square lattice. ( b ) Average d I/ d V spectrum obtained over the region of the sample in a , showing an integrated density of states gap of ~50 meV that sets a minimum value for the band gap at this composition. Setup conditions in: ( a ) I set =10 pA, V set =−100 mV; ( b ) I set =100 pA, V set =−100 mV. Full size image Electronic band structure mapping using LL spectroscopy When a magnetic field is applied perpendicular to the surface of a sample, LLs emerge as peaks in d I/ d V spectra on top of the U-shaped background, which signal the quantization of the two-dimensional surface states ( Fig. 3a,b ). Using a semi-classical approximation, it can be shown that for an isotropic Fermi surface, the magnitude of the momentum vector ( k ) at any given energy E is proportional to ( NB ) 0.5 , where N is the LL index, B is the applied magnetic field and E is the energy of the LL peak. For a non-isotropic Fermi surface, the Fermi surface area is proportional to NB , which can be mapped to an effective (angle-integrated average) momentum given by ( NB ) 0.5 . In either case, this allows us to use LLs to measure the angle-integrated dispersion with high precision. 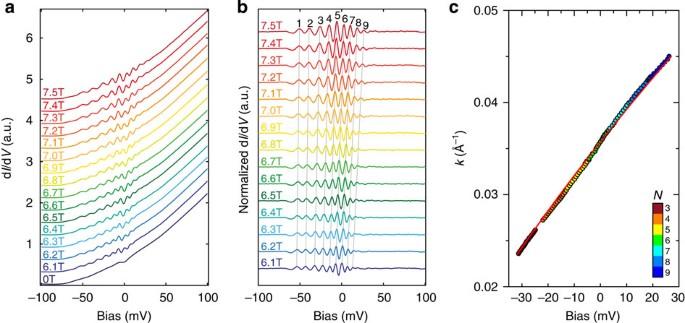Figure 3: LL spectroscopy and the extraction of electronic band dispersion. (a) Average dI/dVspectra, vertically offset for clarity, obtained at different applied magnetic fields. Each spectrum is determined by averaging 64 point-spectra, spaced equally along a 20-nm line cut across the region of the sample shown inFig. 2a. (b) Normalized dI/dVspectra, vertically offset for clarity (seeSupplementary Note 1for normalization details). (c) Average-integrated momentumkversus bias dispersion of a single SS band crossing the Fermi level (circles) and the bare quasiparticle dispersion (red) (Supplementary Note 2). Different colours of circles indicate different LL indices. Setup condition inaare:Iset=100 pA,Vset=−100 mV. Figure 3: LL spectroscopy and the extraction of electronic band dispersion. ( a ) Average d I/ d V spectra, vertically offset for clarity, obtained at different applied magnetic fields. Each spectrum is determined by averaging 64 point-spectra, spaced equally along a 20-nm line cut across the region of the sample shown in Fig. 2a . ( b ) Normalized d I/ d V spectra, vertically offset for clarity (see Supplementary Note 1 for normalization details). ( c ) Average-integrated momentum k versus bias dispersion of a single SS band crossing the Fermi level (circles) and the bare quasiparticle dispersion (red) ( Supplementary Note 2 ). Different colours of circles indicate different LL indices. Setup condition in a are: I set =100 pA, V set =−100 mV. Full size image Our first task is to plot the LL energy as a function of ( NB ) 0.5 . Since precise determination of LL peak positions is of extreme importance for our study, we normalize each d I/ d V spectrum acquired in a magnetic field ( Fig. 3b ) before fitting a Lorentzian curve to locate the position of each LL peak (see Supplementary Fig. 1 and Supplementary Note 1 ). We note that this process is only possible if all d I/ d V spectra are acquired over the ‘identical’ region of the sample with ‘no tip changes’. Next, we index the LLs with integer numbers as shown in Fig. 3b and plot their positions as a function of average-integrated momentum to obtain a continuous dispersion ( Fig. 3c and Supplementary Fig. 2 ). Since the data were acquired in small magnetic field increments of 0.1 T, we are able to obtain nearly 100 data points within the narrow energy range of ±30 meV around the Fermi level. The energy resolution of our experiments is only limited by thermal broadening (~4 k B T , where k B is the Boltzmann constant and T is the temperature) and is ~1.5 meV at 4 K. Extracting the Eliashberg function and mass enhancement factor The real part of the self-energy of the electrons Σ′( k , E ) can be calculated as the difference between the measured dispersion ε ( k ) shown in Fig. 3c and the bare quasiparticle dispersion ε 0 ( k ) ( Fig. 4a ). To get a physical intuition on the bare quasiparticle dispersion, we perform tight-binding calculations on x ~0.09 Pb 1− x Sn x Se to obtain the theoretically predicted surface state (SS) dispersion. As expected, this dispersion is nearly linear with a very small quadratic correction. It can be approximated as a second-degree polynomial in the form of ε 0 ( k )= α ( k − k f )+ β ( k − k f ) 2 , where k f is the momentum wave vector at the Fermi level ( Supplementary Note 2 ). Using coefficients α and β (adjusted by <6% to match our experimental data at energies away from the Fermi level), we can determine Σ′( k , E ) ( Fig. 4a ). The extracted Σ′( k , E ) is antisymmetric with respect to the Fermi level, with positive values for the occupied states and negative values for the unoccupied states. Σ′( k , E ) and the Eliashberg function α 2 F( ω ) are related by the integral equation: , where and f ( x ) is the Fermi distribution function. The inversion of this integral to calculate α 2 F( ω ) is mathematically unstable and results in unphysical solutions [18] . However, this problem can be circumvented by the application of the maximum entropy method (MEM) (ref. 18 ) to fit Σ′( k,E ) and calculate the α 2 F( ω ) of our system ( Fig. 4b and Supplementary Notes 3 and 4 ). In contrast to the use of this method on real self-energy obtained from ARPES [18] , [31] , our measurements allow access to both occupied and unoccupied states, and we can use the whole energy range of these to calculate α 2 F( ω ), thus using more information to converge to the correct α 2 F( ω ). The mass enhancement factor λ is easily calculated from α 2 F( ω ) as . From our data in Fig. 4a , we get λ to be 0.11±0.05. Our measurements reveal weak EPC in this material, which may play a role in the high thermoelectric power observed by other techniques [32] . We note that surface λ measured in our experiments is comparable to the bulk λ reported on similar compounds obtained using Shubnikov–de Haas oscillations [33] . 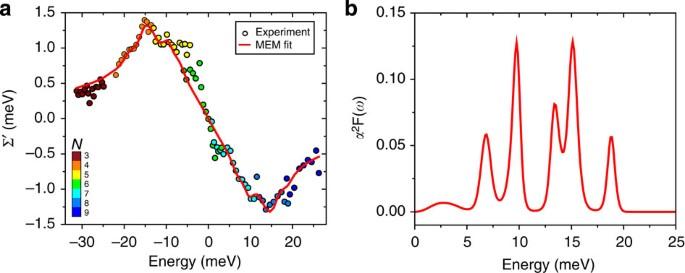Figure 4: Real part of the self-energy (Σ′) and the extraction of the Eliashberg function. (a) Experimentally determined Σ′ (open circles) and the maximum entropy method (MEM) fit (red line). Colours of circles indicate the index of the LL used. (b) The extracted Eliashberg function (red) obtained by using the experimental data ina. Figure 4: Real part of the self-energy (Σ′) and the extraction of the Eliashberg function. ( a ) Experimentally determined Σ′ (open circles) and the maximum entropy method (MEM) fit (red line). Colours of circles indicate the index of the LL used. ( b ) The extracted Eliashberg function (red) obtained by using the experimental data in a . Full size image To demonstrate the validity of our method, we perform the following tests. Both α 2 F( ω ) and λ determined separately using the dispersion of the occupied electronic states ( α 2 F − ( ω ); λ − ) and the unoccupied states ( α 2 F + ( ω ); λ + ) are expected to yield identical results. To check this, we first calculate and directly compare α 2 F − ( ω ) and α 2 F + ( ω ) functions. Remarkably, these two provide an excellent match within our experimental resolution as the principle phonon modes in both are at nearly identical energies ( Supplementary Fig. 3 ), which further confirms the high quality of our experimental data. Moreover, λ − and λ + extracted from curves in Supplementary Fig. 3 are the same within the measurement error. Finally, we apply our method to a second system, Bi 2 Se 3 , to search for the expected signatures of EPC ( Supplementary Note 5 ). Although the reported magnitudes of λ in Bi 2 Se 3 vary widely across different experiments as discussed in the introductory paragraphs, even the smallest detected λ (~0.17 in ref. 13 ) should in principle result in band renormalization large enough to be detected by our novel experimental method. In this endeavour, we use the data from one of the pioneering LL studies in Bi 2 Se 3 acquired in ref. 34 . The extracted SS band dispersion shows a prominent deviation from the smooth evolution noticeable near the Fermi level that clearly signals the presence of EPC ( Supplementary Fig. 4a ). Furthermore, by calculating the real part of the self-energy ( Supplementary Fig. 4b ) we determine λ to be ~0.26, which is within the range of reported values on this material. We note that although the analysis presented here on Bi 2 Se 3 suggests EPC weaker than some of the other studies [14] , [15] , [16] , we cannot exclude the presence of ~3 meV peak reported by Kondo et al . [14] or ~8 meV peak reported by Sobota et al . [16] , and higher resolution future studies may be needed. Nevertheless, the available data and analysis presented here demonstrate yet another confirmation of the validity of our methodology. We expect that this newly developed method of determining EPC by LL spectroscopy will be especially useful for two-dimensional systems like graphene or ultra-thin films as well as in materials where surface states play an important role in determining the electronic properties. In many topological insulators, bulk and surface state electronic bands lie close to each other in energy and momentum and disentangling the two using ARPES can be challenging. Our method provides a natural solution to this problem as the strongly k z -dispersing bulk bands would not be observed using STM, which allows us to examine the effect of phonons exclusively on the topological surface states. Furthermore, phonon modes and EPC itself are likely sensitive to the presence of inhomogeneous structural distortions, and our work provides a way to probe this. For example, ‘stripe’-like inhomogeneity in Bi 2 Te 3 single crystals [28] and surface dislocations in Bi 2 Se 3 thin films [35] have already shown to result in a prominent change in the local density of states, but the evidence of any resulting modification in the phonon spectrum is still lacking. Our new method could provide further insight into the electron–phonon dynamics in these materials at the nanoscale level and could facilitate engineering other novel systems with more desirable properties. How to cite this article: Zeljkovic, I. et al . Nanoscale determination of the mass enhancement factor in the lightly doped bulk insulator lead selenide. Nat. Commun . 6:6559 doi: 10.1038/ncomms7559 (2015).